Protease-degradable electrospun fibrous hydrogels Electrospun nanofibres are promising in biomedical applications to replicate features of the natural extracellular matrix (ECM). However, nearly all electrospun scaffolds are either non-degradable or degrade hydrolytically, whereas natural ECM degrades proteolytically, often through matrix metalloproteinases. Here we synthesize reactive macromers that contain protease-cleavable and fluorescent peptides and are able to form both isotropic hydrogels and electrospun fibrous hydrogels through a photoinitiated polymerization. These biomimetic scaffolds are susceptible to protease-mediated cleavage in vitro in a protease dose-dependent manner and in vivo in a subcutaneous mouse model using transdermal fluorescent imaging to monitor degradation. Importantly, materials containing an alternate and non-protease-cleavable peptide sequence are stable in both in vitro and in vivo settings. To illustrate the specificity in degradation, scaffolds with mixed fibre populations support selective fibre degradation based on individual fibre degradability. Overall, this represents a novel biomimetic approach to generate protease-sensitive fibrous scaffolds for biomedical applications. An increased understanding of the contributions of extracellular matrix (ECM) structural features (for example, fibre size and orientation) in guiding tissue function has motivated researchers to create biomimetic scaffolds with increased structural complexity [1] . In particular, three methods—self-assembly [2] , [3] , phase separation [4] , [5] and electrospinning [6] , [7] —have emerged as techniques to generate fibrous scaffolds with electrospinning becoming the most ubiquitous method due to its ease of set-up, scalability and feasibility with a diverse array of polymers. A wide variety of natural and synthetic polymers have been electrospun and demonstrated utility in various biomedical applications including vascular grafts [8] , drug delivery [9] , contraception and sexually transmitted disease prevention [10] , and cardiac [11] , [12] , skeletal [13] , [14] , dermal [15] and craniofacial [16] tissue formation. Together, these and other studies have indicated that scaffold structural features can influence cell morphology [14] , alignment [17] , migration [18] , differentiation [19] and tissue organization [13] . Despite the success of these materials in replicating the anisotropic, fibrous structure of natural ECM, the majority of electrospun materials are synthetic (non-bioactive) and hydrophobic and/or semi-crystalline (that is, polycaprolactone, poly(lactic acid), poly(lactic-co-glycolic acid)) such that fibres are rigid with limited water absorption, in stark contrast to the bioactive, flexible, hydrated state of natural ECM. Moreover, these electrospun scaffolds are either non-degradable or degrade hydrolytically, through passive release determined by material crystallinity, hydrophobicity and stability of the polymer backbone to hydrolysis. Meanwhile, natural ECM components are bioactive and degrade proteolytically, through dynamic interactions with matrix metalloproteinases (MMPs) that are actively regulated in natural ECM remodelling [20] , [21] . As an alternative to synthetic polymers, components of natural ECM such as proteins have also been electrospun [22] . Since Matthews et al . [23] electrospun Type I and Type III collagen in 2002, other natural proteins such as other types of collagen [24] , gelatin [25] , fibrinogen [26] and elastin [24] have been electrospun. These electrospun scaffolds exhibit some level of bioactivity, mimic features of the flexible, hydrated state of natural soft-tissue microenvironments and may be enzymatically degradable due to their primary amino acid sequence [22] . However, these hydrophilic scaffolds require crosslinking to stabilize the structural features of the scaffold on introduction to aqueous environments. This crosslinking with gluteraldehyde [27] or other agents [22] may present toxicity issues, and modifications of the natural polymers (for example, crosslinking of amines) may limit their bioactivity. Not surprisingly, electrospinning may damage secondary and higher order protein structure such that only ~42% of the characteristic spacing between each polyproline-II helix of natural collagen is retained after electrospinning [28] . Structural differences between natural and electrospun proteins are further compounded by batch-to-batch variations of proteins purified from animal sources [29] . From an engineering view, perhaps the most striking limitation of electrospun natural proteins is the limited ability to alter many of their properties, including enzymatic degradation. The primary amino acid sequence and conformation of the protein dictates the rate of enzymatic cleavage, neither of which may be effectively controlled through electrospinning. Isotropic hydrogels have been synthetically crosslinked with protease-degradable peptides to combine the benefits of enzymatic degradability with material tunability [30] , [31] , [32] , [33] , [34] , [35] . Studies have illustrated that this protease-mediated degradation is an important regulator in bone formation [30] , angiogenesis [31] , and tissue function after myocardial infarction [35] . However, the chemistry and crosslinking used in these studies relies on spontaneous gelation after mixing reagents and is not compatible with electrospinning; thus, proteases-sensitive degradation has not yet been translated to synthetic fibrous hydrogels. Here we report an approach to create protease-degradable electrospun hydrogels through chemical modification of hyaluronic acid (HA—a linear polysaccharide composed of alternating D-glucuronic acid and N -acetyl-D-glucosamine), combining the bioactivity of a natural polymer with the importance of engineered enzymatic sensitivity. We demonstrate that isotropic hydrogels and electrospun hydrogels crosslink through photopolymerizable peptides and swell on hydration. In vitro and in vivo , scaffold degradation behaviour in the presence of exogenously added or natural proteases varies when a protease-degradable or non-degradable peptide is incorporated. To our knowledge, this approach represents the first electrospun hydrogel that degrades through engineered protease sensitivity. Design of protease-sensitive photocrosslinkable HA HA was chosen as the primary macromer component because it is a bioactive molecule of natural ECM and is microbially sourced to limit purification concerns associated with ECM proteins sourced from animals. Furthermore, HA has a repeat structure with several functional groups (for example, hydroxyls and carboxyls) amenable to chemical modification and may contain several hundred repeat units to enable varying degrees of functionalization [36] . Previous studies have also successfully electrospun methacrylate-functionalized HA into scaffolds consisting of stable, water-swollen fibres that mimic the microenvironments of many soft tissues [37] . Conceptually, we hypothesized that by incorporating a protease-degradable or non-degradable sequence between the methacrylate group and HA backbone, we could generate a starting material that would crosslink through methacrylates and degrade through the specificity of the designed peptide sequence. With this goal in mind, we took a modular approach to macromer synthesis consisting of three steps—synthetic modification of HA with maleimides, synthesis of methacrylated peptides (MePs) and fluorophore peptides with terminal thiols as nucleophiles for Michael addition, and modular attachment of peptides via thiol-maleimide Michael addition. In the first step, maleimide HA (MaHA) was synthesized by reacting aminated maleimide salt with tetrabutylammonium-HA (soluble in organics) via a BOP ((Benzotriazol-1-yloxy)tris(dimethylamino)phosphonium hexafluorophosphate) coupling agent to form an amide linkage between the carboxyl group of HA and the amine group of the maleimide salt ( Fig. 1a , Supplementary Fig. 1 ). Maleimides are known to undergo near quantitative, rapid (seconds−minutes) click reactions with thiols that allows for efficient conjugation of photopolymerizable peptides [38] . Compared with previously reported esterification modifications of HA [34] , the amide linkage between the maleimide group and HA was chosen to limit hydrolysis of the linkage after peptide conjugation. 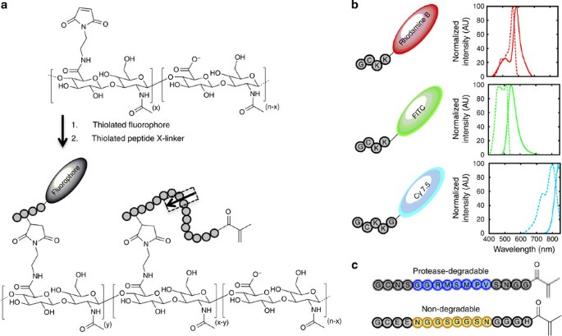Figure 1: Synthesis and molecular design of macromer components. (a) Schematic of modular MePHA synthesis from the combination of maleimide HA (MaHA—top) and thiolated peptides (fluorophores or crosslinkers). Protease-degradable MePHA (bottom) contains a protease-mediated cleavage site (dotted rectangle) to facilitate degradation while the fluorophore facilitates monitoring of degradation andin situimaging. (b) Thiolated peptide fluorophores (amino acids sequences listed in circles) synthesized via solid-phase synthesis to covalently label MePHA and their corresponding excitation (dotted lines) and emission (solid lines) spectra. (c) Thiolated peptide crosslinkers designed to contain a thiol at one end (cysteine), a central sequence sensitive to protease degradation (blue) or insensitive to protease degradation (orange), and a photopolymerizable end group (methacrylate) to permit ultraviolet light-initiated polymerization. Figure 1: Synthesis and molecular design of macromer components. ( a ) Schematic of modular MePHA synthesis from the combination of maleimide HA (MaHA—top) and thiolated peptides (fluorophores or crosslinkers). Protease-degradable MePHA (bottom) contains a protease-mediated cleavage site (dotted rectangle) to facilitate degradation while the fluorophore facilitates monitoring of degradation and in situ imaging. ( b ) Thiolated peptide fluorophores (amino acids sequences listed in circles) synthesized via solid-phase synthesis to covalently label MePHA and their corresponding excitation (dotted lines) and emission (solid lines) spectra. ( c ) Thiolated peptide crosslinkers designed to contain a thiol at one end (cysteine), a central sequence sensitive to protease degradation (blue) or insensitive to protease degradation (orange), and a photopolymerizable end group (methacrylate) to permit ultraviolet light-initiated polymerization. Full size image Second, thiolated peptides (containing a cysteine amino acid) were synthesized with terminal methacrylate groups or fluorophores by adding methacrylic acid or carboxylated fluorophores (Rhodamine B, 5(6)-Carboxyfluorescein (FITC) and Cyanine7.5), respectively, as the terminal reactant in solid-phase peptide synthesis ( Fig. 1b,c ). Thiolated fluorophores (GCKK-Rho, GCKK-FITC and GCKKG-Cyanine7.5) were synthesized to directly label HA with fluorescent dyes to accurately quantify HA erosion from scaffolds in vitro (GCKK-Rho and GCKK-FITC) and in vivo (GCKKG-Cyanine7.5); therefore, their excitation and emission spectra were analysed to aid in subsequent fluorometric spectroscopy ( Fig. 1b ). The protease-degradable peptide ( Fig. 1c ) was based on previous studies that indicated enhanced susceptibility to MMP-1 and MMP-2 mediated cleavage within the central 8 amino acid sequence [31] . The non-degradable peptide ( Fig. 1c ) is a novel sequence that was designed to be resistant to degradation by numerous enzymes (that is, MMPs, pepsin and trypsin) and contain the same number of amino acids as the protease-degradable peptide to aid in comparisons between the two sequences. To evaluate the proteolytic sensitivity, peptides were placed at varying concentrations into recombinant human MMP-2 (rhMMP-2) or Type II collagenase (broad range of proteases) to determine the kinetic parameters for protease-mediated cleavage using a modified fluorescamine assay [30] , [31] , [39] . The protease-degradable peptide followed Michaelis–Menten kinetics ( Table 1 , Supplementary Fig. 2 ) in rhMMP-2 and collagenase and had kinetic parameters similar to those previously reported in rhMMP-2 (ref. 31 ); however, the non-degradable peptide kinetic parameters were not measurable as cleavage was not detectable for the duration of the assay (9 h). Table 1 Kinetic parameters for peptide crosslinkers. Full size table In the final step, peptides were conjugated to MaHA by first mixing thiolated fluorophores with MaHA to consume a small portion of maleimides. Next, excess MeP was added to consume all remaining maleimide groups, and the product was dialyzed and lyophilized to yield the macromer Methacrylated Peptide HA (MePHA, Fig. 1a ). For consistency, GCKK-Rho was conjugated to all non-degradable MePHA (crosslinks through non-degradable peptide) and GCKK-FITC to all protease-degradable MePHA (crosslinks through protease-degradable peptide) for all subsequent in vitro characterization. GCKKG-Cyanine7.5 was conjugated to both protease-degradable and non-degradable MePHA used in vivo . Isotropic hydrogel formation and characterization After MePHA synthesis, isotropic, non-fibrous hydrogels were fabricated to evaluate the sensitivity of the different MePHA formulations (protease degradable and non-degradable) to enzyme-mediated degradation. Furthermore, the formation of isotropic hydrogels allows for comparison to previous reports of non-fibrous, protease-degradable hydrogels [30] , [31] , [35] , [40] , [41] . Isotropic MePHA hydrogels were formed as 4 or 2 wt% cylindrical discs via ultraviolet-mediated radical crosslinking with Irgacure 2959 (I2959) as a radical photoinitiator in TTC buffer (Tris, Triton X-100, CaCl 2 ). To ensure similar mechanical properties between different MePHA formulations, storage moduli were measured by oscillatory rheology. Protease-degradable hydrogels at 2 wt% (250±14 Pa) and 4 wt% (1.18±0.46 kPa) showed no statistical differences between moduli of equivalent hydrogels of non-degradable MePHA at 2 wt% (300±60 Pa) and 4 wt% (1.51±0.08 kPa), indicating similar gelation between different MePHA formulations ( Supplementary Fig. 3 ). For degradation studies, MePHA hydrogels were incubated in TTC buffer for 48 h at 37 °C and retained their cylindrical shape ( Fig. 2a,b ). Hydrogels were subsequently placed into varying concentrations of Type II collagenase (1 to 500 U ml −1 ), rhMMP-2 (5 nM) or TTC buffer and monitored for HA release. Collagenase contains a broad range of MMPs and facilitates general comparison with previous reports of protease-degradable hydrogels eroded with collagenase [33] , [41] . Alternatively, rhMMP-2 was chosen to assess degradation in the presence of a specific MMP at a concentration that is indicative of previously reported physiologic concentrations (1–20 nM) [42] , [43] , [44] , [45] . 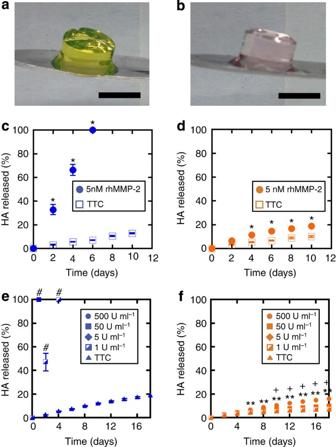Figure 2:In vitroisotropic MePHA hydrogel degradation. Non-fibrous hydrogels of protease-degradable (a) and non-degradable (b) MePHA equilibrated for 48 h at 37 °C retain their cylindrical shape. Scale bar, 5 mm. (c–f) Quantification of HA release from 2 wt% MePHA hydrogels crosslinked with protease-degradable (c,e) or non-degradable (d,f) methacrylated peptides in 5 nM rhMMP-2 (c,d), varying concentrations of Type II collagenase ((e,f) listed in units of activity per ml) or TTC buffer. Media (rhMMP-2, collagenase or TTC buffer) was refreshed every 2 days to maintain enzyme activity and HA release was quantified by monitoring release of a fluorophore covalently bonded to HA. Error bars represent s.d. (n=3, 4). *P<0.05 versus TTC. #—all isotropic protease-degradable hydrogels degraded in Type II collagenase were statistically different from control (TTC) at all time points,P<0.05. **P<0.05 500 U ml−1versus TTC, +P<0.05 50 U ml−1versus TTC. Figure 2: In vitro isotropic MePHA hydrogel degradation. Non-fibrous hydrogels of protease-degradable ( a ) and non-degradable ( b ) MePHA equilibrated for 48 h at 37 °C retain their cylindrical shape. Scale bar, 5 mm. ( c – f ) Quantification of HA release from 2 wt% MePHA hydrogels crosslinked with protease-degradable ( c , e ) or non-degradable ( d , f ) methacrylated peptides in 5 nM rhMMP-2 ( c , d ), varying concentrations of Type II collagenase (( e , f ) listed in units of activity per ml) or TTC buffer. Media (rhMMP-2, collagenase or TTC buffer) was refreshed every 2 days to maintain enzyme activity and HA release was quantified by monitoring release of a fluorophore covalently bonded to HA. Error bars represent s.d. ( n =3, 4). * P <0.05 versus TTC. #—all isotropic protease-degradable hydrogels degraded in Type II collagenase were statistically different from control (TTC) at all time points, P <0.05. ** P <0.05 500 U ml −1 versus TTC, + P <0.05 50 U ml −1 versus TTC. Full size image Isotropic protease-degradable MePHA hydrogels eroded (that is, 100% of HA released) within a day to up to 6 days in response to rhMMP-2 and varying collagenase concentration ( Fig. 2c,e , Supplementary Fig. 4 ). These rhMMP-2 and collagenase-dependent degradation rates agree with previously reported isotropic HA hydrogels crosslinked via addition of MMP-sensitive di-thiol peptides [41] . When incubated in buffer, isotropic protease-degradable MePHA hydrogels retained >80% of their original HA content after 18 days, demonstrating the stability of the hydrogel to non-enzymatic degradation. Conversely, all non-degradable MePHA hydrogels retained >80% of their original HA content, irrespective of the presence of rhMMP-2 or concentration of collagenase within the tested range ( Fig. 2d,f , Supplementary Fig. 4 ). Together with the kinetic parameters of the individual MePs, this result further indicates that erosion of these hydrogels occurs through protease-mediated cleavage of the peptide crosslinker. Notably, previous erosion studies of hydrogels crosslinked with amino acid sequences insensitive to protease-mediated cleavage were completed in low concentrations of specific recombinant MMPs [30] , [31] , whereas the study reported here also demonstrates resistance to enzyme-mediated degradation in high concentrations of a broad range of proteases. Electrospun fibrous hydrogel formation and characterization To generate electrospun fibrous hydrogels, solutions of MePHA (1 wt%) and polyethylene oxide (PEO; 4.5 wt%) were mixed with I2959 in TTC buffer and electrospun as thin films (10–30 μm) on methacrylated coverslips (for optical microscopy) or as standalone mats (~1-mm dry thickness, for in vitro degradation studies) ( Fig. 3a ). Electrospun scaffolds were exposed to ultraviolet light to initiate radical crosslinking ( Fig. 3a ) and then further crosslinked with additional light exposure after hydration to stabilize fibres in their swollen state. Aqueous solutions of HA have a relatively high surface tension at low HA concentrations, which limits molecular entanglement and the ability to form smooth electrospun nanofibres [46] ; therefore, PEO was included as a bioinert, hydrophilic polymer to increase molecular chain entanglement at lower HA concentrations to improve fibre morphology. 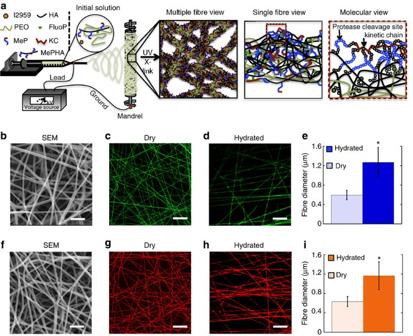Figure 3: Electrospun fibrous MePHA hydrogel characterization. (a) Schematic of electrospinning and molecular composition of MePHA fibrous scaffolds. Molecular view highlights the sites of protease cleavage and kinetic chain formation between methacrylated peptides after crosslinking. FluoP, fluorescent peptide; KC, kinetic chain. Representative SEM images of protease-degradable (b) and non-degradable (f) electrospun MePHA. Fluorescent confocal microscopy images of protease-degradable (c,d) and non-degradable (g,h) electrospun MePHA scaffolds in the dry and hydrated states. (e,i) Quantification of fibre diameters before (dry) and after swelling (hydrated) from confocal images of protease-degradable (e) and non-degradable (i) MePHA scaffolds. Error bars represent s.d. *P<0.05. Scale bars,b,f—2 μm,c,d,g,h—25 μm. Figure 3: Electrospun fibrous MePHA hydrogel characterization. ( a ) Schematic of electrospinning and molecular composition of MePHA fibrous scaffolds. Molecular view highlights the sites of protease cleavage and kinetic chain formation between methacrylated peptides after crosslinking. FluoP, fluorescent peptide; KC, kinetic chain. Representative SEM images of protease-degradable ( b ) and non-degradable ( f ) electrospun MePHA. Fluorescent confocal microscopy images of protease-degradable ( c , d ) and non-degradable ( g , h ) electrospun MePHA scaffolds in the dry and hydrated states. ( e , i ) Quantification of fibre diameters before (dry) and after swelling (hydrated) from confocal images of protease-degradable ( e ) and non-degradable ( i ) MePHA scaffolds. Error bars represent s.d. * P <0.05. Scale bars, b , f —2 μm, c , d , g , h —25 μm. Full size image Electrospun scaffolds were characterized by unconfined compression testing and by scanning electron microscopy (SEM; dry scaffolds) and confocal microscopy (dry and hydrated scaffolds) to investigate fibre morphology, diameter and swelling behaviour. Similar bulk compressive moduli were observed in protease-degradable (2.8±1.0 kPa) and non-degradable (3.4±0.7 kPa) MePHA scaffolds. Meanwhile, SEM indicated smooth fibre morphology throughout scaffolds and submicron diameters for both protease-degradable (320±100 nm) and non-degradable (270±60 nm) MePHA scaffolds ( Fig. 3b,f , Supplementary Fig. 5 ). When analysing fibre morphology and diameter in the dehydrated state, artifacts may be introduced in SEM during drying (for example, alcohol dehydration, flash freezing/lyophilization and critical point drying). Consequently, fibre diameters of fluorescently labelled dry and hydrated scaffolds were also measured in situ using confocal microscopy to determine the degree of fibre swelling ( Fig. 3c–e,g–i ). Protease-degradable MePHA fibre diameters increased from 590±100 nm before hydration to 1.27±0.31 μm at equilibrium swelling, and non-degradable MePHA fibre diameters increased similarly from 640±100 nm before hydration to 1.17±0.29 μm at equilibrium swelling. Scaffold porosity was also quantified by confocal microscopy and indicated high porosity in both protease-degradable (82±4%) and non-degradable (79±4%) MePHA scaffolds. No significant differences existed between bulk compressive modulus, fibre diameters or porosity of protease-degradable and non-degradable MePHA, demonstrating that both electrospun hydrogels display similar mechanical properties and swelling behaviour. To investigate the enzyme-mediated degradation of electrospun protease-degradable and non-degradable MePHA, fibrous scaffolds were placed into TTC buffer, rhMMP-2 (10 nM) or Type II collagenase (5–500 U ml −1 ) and HA release was monitored ( Fig. 4a,e , Supplementary Fig. 6 ). Protease-degradable MePHA scaffolds showed a collagenase concentration-dependent burst release of degradation products within the first 48 h, with >80% of HA released from the networks across all collagenase concentrations at 2 weeks; however, in the absence of collagenase these scaffolds retained over 75% of MePHA content after 3 weeks ( Fig. 4a ). In comparison, non-degradable MePHA scaffolds all retained >75% of MePHA content after 3 weeks, regardless of collagenase concentration ( Fig. 4e ), showing similar degradation profiles to those observed in isotropic, non-fibrous hydrogels ( Fig. 2d ). Similar trends were also observed in rhMMP-2 as protease-degradable scaffolds released nearly 30% of HA after 8 days compared with 6% release of HA in non-degradable scaffolds ( Supplementary Fig. 6 ). Interestingly, all protease-degradable scaffolds degraded more rapidly at early time points but slowed in degradation at later time points. HA release from protease-degradable MePHA at later time points in collagenase and rhMMP-2 was greater than the passive release observed in TTC buffer, suggesting that protease-mediated degradation was still occurring within the scaffolds for the duration of the study, albeit at slower rates. 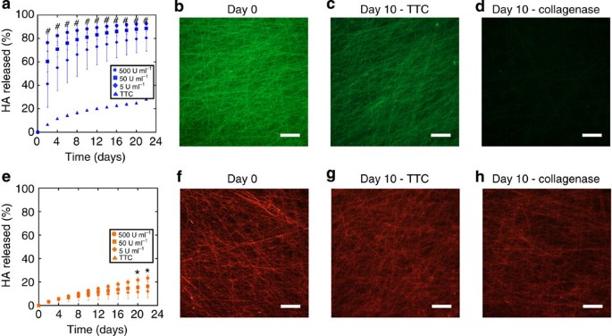Figure 4:In vitrofibrous MePHA hydrogel degradation. HA release profiles of electrospun protease-degradable (a) or non-degradable (e) MePHA scaffolds in varying concentrations of Type II collagenase (listed in units of activity per ml) or TTC buffer. HA release was quantified by monitoring release of a fluorophore covalently bonded to HA. Error bars represent s.d. #—all protease-degradable scaffolds in Type II collagenase (500–5 U ml−1) were statistically different from control (TTC) at all time points (2–22 days),P<0.05. *P<0.05 500 U ml−1versus TTC. (b–d,f–h) Representative wide-field fluorescent microscopy images of thin film electrospun protease-degradable (b–d) or non-degradable (f–h) MePHA scaffolds at day 0 (b,f) and after incubation at 37 °C in TTC buffer (c,g) or 500 U ml−1Type II collagenase (d,h) for 10 days. Media (collagenase or TTC buffer) was refreshed every 2 days for all scaffolds to maintain enzyme activity. Scale bars, 100 μm. Figure 4: In vitro fibrous MePHA hydrogel degradation. HA release profiles of electrospun protease-degradable ( a ) or non-degradable ( e ) MePHA scaffolds in varying concentrations of Type II collagenase (listed in units of activity per ml) or TTC buffer. HA release was quantified by monitoring release of a fluorophore covalently bonded to HA. Error bars represent s.d. #—all protease-degradable scaffolds in Type II collagenase (500–5 U ml −1 ) were statistically different from control (TTC) at all time points (2–22 days), P <0.05. * P <0.05 500 U ml −1 versus TTC. ( b – d , f – h ) Representative wide-field fluorescent microscopy images of thin film electrospun protease-degradable ( b – d ) or non-degradable ( f – h ) MePHA scaffolds at day 0 ( b , f ) and after incubation at 37 °C in TTC buffer ( c , g ) or 500 U ml −1 Type II collagenase ( d , h ) for 10 days. Media (collagenase or TTC buffer) was refreshed every 2 days for all scaffolds to maintain enzyme activity. Scale bars, 100 μm. Full size image To ensure that the chemical structure of the protease-degradable peptide was not damaged by ultraviolet exposure during crosslinking (thus altering the sensitivity of the peptide), methacrylated protease-cleavable peptides were exposed to equivalent ultraviolet treatment and analysed via matrix-assisted laser desorption ionization—time of flight mass spectroscopy (MALDI–TOF). No changes in molecular weight with ultraviolet exposure were observed ( Supplementary Fig. 7 ). To ensure the profiles were not the result of fluorophore cleavage from the HA backbone, degradation was also analysed via uronic acid assay ( Supplementary Fig. 8 ), confirming the same general profile observed via fluorometric analysis. Previous models of hydrolytic degradation of hydrogels formed through multi-vinyl crosslinks [47] indicate that at early time points, erosion occurs primarily through release of the crosslinking molecule from the network, followed by a plateau of degradation products until kinetic chains are finally released very late on reverse gelation. The erosion of the protease-degradable electrospun MePHA scaffolds reported here follows a similar profile, suggesting that HA release (crosslinking molecule) dominates the initial degradation profile with a corresponding general plateau in degradation rate at later time points until all kinetic chains are released from the network. To observe fibre degradation in situ , thin films of fluorescent protease-degradable and non-degradable MePHA were attached to methacrylated glass slides and imaged at different times within collagenase (500 U ml −1 ) or TTC buffer ( Fig. 4b–d,f–h ). Similar to the trends observed in free-swelling mats, protease-degradable MePHA fibres eroded in collagenase but remained stable in TTC buffer, while all non-degradable MePHA scaffolds remained intact for the duration of the study. To further visualize fibre degradation, multi-fibre scaffolds were created by co-electrospinning separate solutions of protease-degradable and non-degradable MePHA ( Fig. 5a ). This process generates fibrous hydrogels with biphasic (protease-mediated and passive) degradation and permits visualization of protease-degradable and non-degradable fibre erosion within the same scaffold ( Fig. 5b,c ). Accordingly, we observed enzyme-mediated degradation of the protease-degradable fibres, whereas non-degradable fibres retained their structure after 10 days of incubation in collagenase (500 U ml −1 ). 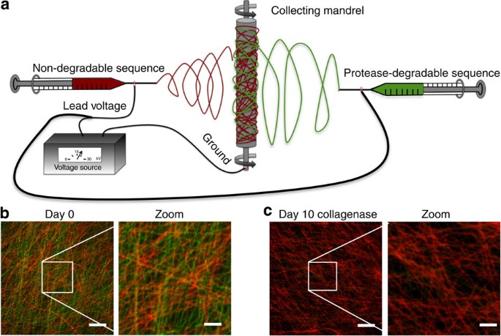Figure 5: Co-electrospun fibrous MePHA hydrogel scaffolds. (a) Schematic of co-electrospinning set-up to form fibrous scaffolds that contain both protease-degradable (green) and non-degradable (red) MePHA fibres. (b,c) Representative wide-field fluorescent microscopy images of co-electrospun MePHA at day 0 (b) and after 10 days of incubation at 37 °C in 500 U ml−1Type II collagenase (c). Media (collagenase or TTC buffer) was refreshed every 2 days to maintain enzyme activity. Scale bars, 100 μm, zoom—25 μm. Figure 5: Co-electrospun fibrous MePHA hydrogel scaffolds. ( a ) Schematic of co-electrospinning set-up to form fibrous scaffolds that contain both protease-degradable (green) and non-degradable (red) MePHA fibres. ( b , c ) Representative wide-field fluorescent microscopy images of co-electrospun MePHA at day 0 ( b ) and after 10 days of incubation at 37 °C in 500 U ml −1 Type II collagenase ( c ). Media (collagenase or TTC buffer) was refreshed every 2 days to maintain enzyme activity. Scale bars, 100 μm, zoom—25 μm. Full size image In vivo erosion of electrospun scaffolds was investigated by covalently attaching a near-infrared (NIR) peptide dye (GCKKG-Cyanine7.5) to MePHA, subcutaneously implanting scaffolds in a murine model and monitoring the corresponding loss in signal intensity over a 6-week period ( Fig. 6 ). Protease-degradable MePHA scaffolds demonstrated faster erosion in vivo over the first 3 weeks (losing nearly 50% of the NIR signal) with considerably slower erosion thereafter. Thus, the in vivo erosion follows a similar trend to in vitro degradation profiles, with the fastest rates of degradation at earlier times and progressively slower degradation at later times. Relative protease levels may also contribute to the observed in vivo erosion profile since MMP activity is known to increase during natural ECM remodelling immediately following tissue injury [42] . It is worth noting that in vivo erosion requires degradation and clearance of HA from the tissue, whereas in vitro degradation is monitored in an aqueous environment with fewer diffusion barriers to HA release from the network. In comparison to protease-degradable MePHA scaffolds, non-degradable MePHA scaffolds eroded at a more linear rate and retained greater HA content throughout the duration of the study, further offering evidence that proteases mediate the observed degradation of protease-degradable MePHA scaffolds in vivo . It was not possible to identify distinct scaffold margins histologically, as the scaffolds were encompassed within cellular tissue for both protease-degradable and non-degradable formulations ( Supplementary Fig. 9 ). Notably, the differences in degradation between protease-degradable and non-degradable MePHA in vitro were not as pronounced in the subcutaneous in vivo model. The observed differences may be due to several factors including supra-physiological protease levels, the absence of protease inhibitors, and limited barriers to diffusive release of HA in vitro . In comparison, mechanical stimulation, blood flow perfusion, cell release of soluble and insoluble signals, and clearance from the site of implantation will influence in vivo degradation. 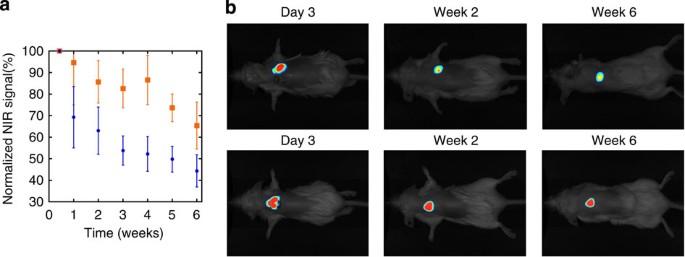Figure 6:In vivofibrous MePHA hydrogel degradation. (a) Erosion of protease-degradable (blue circles) and non-degradable (orange squares) electrospun fibrous MePHA in a subcutaneous mouse model quantified by signal decay of a Cyanine7.5 dye covalently bonded to HA before scaffold formation. Error bars represent s.e. (n=4, 3). (b) Representative serialin vivooptical images used to quantify HA release from the site of implantation. Figure 6: In vivo fibrous MePHA hydrogel degradation. ( a ) Erosion of protease-degradable (blue circles) and non-degradable (orange squares) electrospun fibrous MePHA in a subcutaneous mouse model quantified by signal decay of a Cyanine7.5 dye covalently bonded to HA before scaffold formation. Error bars represent s.e. ( n =4, 3). ( b ) Representative serial in vivo optical images used to quantify HA release from the site of implantation. Full size image Fibrous hydrogels are gaining widespread attention in biomedical applications due to their ability to mimic many features of the ECM; however, most fibre systems are either rigid polymers that lack sensitivity to enzymes or are natural polymers with disrupted biological activity during processing or limited sourcing. Current strategies that focus on engineering protease-sensitive surface coatings [48] or protease-sensitive surface linkers [49] do not allow for the electrospun network itself to degrade in response to proteases. To address these limitations, we developed a generalizable chemical scheme to formulate fluorescently labelled HA macromers that can be electrospun and then crosslinked through MePs and degrade through the sensitivity of the incorporated amino acid sequence. In particular, this approach permits material crosslinking in the dry state so that electrospun fibrous structures may be stabilized after scaffold formation. In contrast, common chemical schemes that crosslink hydrogels through addition reactions between peptides and a functionalized polymer (that is, four-arm or eight-arm PEG) [31] , [50] must be performed in a hydrated state; therefore, they do not translate to electrospinning processes. Two photopolymerizable, protease-degradable macromers have been synthesized previously, namely, acrylate-PEG-(peptide-PEG) m -acrylate [40] and acrylate-peptide-PEG-peptide-acrylate [33] ; however, the former contains a high molecular weight between crosslinks (500 kDa) that may limit its ability to form stable fibres, while the latter contains a considerably lower molecular weight between crosslinks (6.4 kDa) that may limit electrospinning and would require very high concentrations of to crosslink. In comparison, our approach has a low average molecular weight between reactive groups (~15 kDa) and a large molecular weight (~140 kDa) to permit stable crosslinking of fibres. Although the scheme reported here used HA, the approach of grafting MePs to a polymer via thiol-maleimide Michael addition is amenable to other polysaccharides or hydrophilic synthetic polymers. The modular approach presented here further allows for conjugating other amino acids of interest to enhance bioactivity through cell adhesive amino acid sequences such as arginine-glycine-aspartic acid (RGD, derived from fibronectin). Another benefit to this system is the ability to electrospin from a non-organic solvent so that growth factors or other soluble signals may be incorporated within fibres for enzyme-mediated release from the network. This release may also be made biphasic by generating a co-electrospun scaffold of protease-degradable and non-degradable MePHA ( Fig. 5a ), where individual fibre degradation is controlled through the degradation of that fibre. Enzymatically mediated selective erosion could be beneficial in controlling release of the network in response to temporal changes in the microenvironment like those observed in the immune response or during wound healing [20] . As a fibrous hydrogel, the system is best suited to soft-tissue applications and may not be suitable for load bearing tissue applications (for example, musculoskeletal). Importantly, this work represents the introduction of protease-mediated degradation as a mechanism for erosion in electrospun fibrous hydrogels. Previous reports have demonstrated protease-mediated degradation in fibrous scaffolds of self-assembling peptide amphiphiles (PAs) designed to contain an MMP-cleavable central domain [51] and in β-sheet forming multidomain peptides with a central three amino acid MMP-cleavable motif [52] . These reports have shown that MMP-cleavable PAs lose 70% of their mass at 2 weeks in 2 mg ml −1 collagenase (Type IV) [51] , and that β-sheet forming multidomain peptides lose 95% of their mass at 2 weeks in 3 mg ml −1 collagenase (Type IV) [52] . While our studies were conducted in a different type collagenase (Type II-higher tryptic levels), the electrospun scaffolds reported here lose 75% mass at 2 weeks in significantly lower concentrations of collagenase, 0.015 mg ml −1 (5 U ml −1 —Type II). Self-assembling peptides and PAs are beneficial for their ability to generate nanoscale diameters (~6–8 nm) and their ability to form in situ , making them an attractive platform as injectable fibrous materials [51] , [52] ; however, mechanical robustness and complex design, synthesis and scalability may limit their widespread use. Conversely, electrospun scaffolds have significantly larger fibre diameters and are not directly injectable; yet, the technique is easy to set-up, scalable and applicable to many polymers. Therefore, incorporating protease-mediated degradation into electrospun scaffolds with a generalizable approach may be translatable to a number of materials and applications. Despite the widespread use of electrospun scaffolds in biomedical applications and the importance of protease-mediated cleavage in biological processes, engineered protease degradation is yet to be explored in electrospun hydrogels. This report makes use of a modular approach to generate electrospinnable macromers that degrade through peptide crosslinks and demonstrates their in vitro degradation and in vivo erosion profiles. These results present a novel degradation mechanism for engineered electrospun hydrogels, an approach that may benefit in vitro and in vivo investigations by synthetic inclusion of biochemically relevant degradation within biophysically relevant scaffolds. Solid-phase peptide synthesis All materials are from Sigma-Aldrich unless noted otherwise. Protease-degradable peptide (GCNS- GGRM↓ SMPV -SNGG-Methacrylate), non-degradable peptide (GCEE-NGGSGGSN-GGGH-Methacrylate) and thiolated peptide fluorophores (GCKK-FITC, GCKK-Rhodamine and GCKKG-Cyanine7.5) were each synthesized with a thiol to facilitate Michael addition coupling to MaHA. The protease-degradable sequence is listed in italics where protease-mediated cleavage is known to occur at the indicated arrow, between the central serine and methionine amino acids. Briefly, peptides were synthesized on Glycinol 2-Chlorotrityl resin (protease-degradable, non-degradable, GCKKG-Cyanine7.5) (Novabiochem) or 1,6-Diaminohexane trityl resin (GCKK-FITC, GCKK-Rhodamine) (Novabiochem) using a PS3 automated solid-phase peptide synthesizer (Protein Technologies, Inc.) via standard FMOC chemistry. The resin was deprotected with 20% (v/v) piperidine in N,N-dimethylformamide, and FMOC-protected amino acids (Novabiochem) were then activated with HBTU (Novabiochem) and 0.4 M methylmorpholine in N,N-dimethylformamide before being added to the reaction vessel four times excess to resin functional groups. To add non-amino acid terminal functional groups to the peptides, the corresponding carboxylic acid form of the functional group (methacrylic acid, 5(6)-carboxyflourescein, Rhodamine B or Cyanine7.5 carboxylic acid (Lumiprobe)) was added in the last step of synthesis. Peptides were cleaved in a 10 ml solution of 95% trifluoroacetic acid, 2.5% triisopropylsilane and 2.5% DI H 2 O, precipitated twice in cold diethyl ether (−80 °C) and allowed to dry overnight. Peptides were dissolved in deionized (DI) H 2 O, flash frozen in liquid nitrogen, lyophilized and stored under nitrogen at −20 °C until use or analysed for purity by MALDI–TOF to confirm synthesis ( Supplementary Figs 10,11 ). Protease-degradable and non-degradable peptides were further analysed via 1 H NMR (Bruker DMX 360 MHz) and the degree of methacrylation per peptide was determined (~100%) by calibrating to known amino acid peaks for valine (protease-degradable sequence) or histidine (non-degradable sequence) ( Supplementary Fig. 12 ). Thiolated fluorophore excitation and emission spectra were measured using a Tecan Spectrometer ( Fig. 1b ). Degradation kinetics Kinetic parameters for protease-degradable and non-degradable peptides were measured using a modified fluorometric assay as previously published [30] , [39] . Briefly, peptides (50–500 μM) were incubated with 1 U ml −1 Type II Collagenase (Worthington Biochemical) or 1 nM rhMMP-2 (R&D Systems) in fluorescence buffer (50 mM tricine, 50 mM NaCl, 10 mM CaCl 2 , 0.05% Brij-35, pH 7.4) at 37 °C. Substrate cleavage was monitored by reacting 20 μl fluorescamine (50 mM in acetone) with 75 ml of substrate/enzyme solution and detecting fluorescence (excitation: 380 nm, emission: 480 nm) on a Tecan Spectrometer. Initial reaction velocities were determined from plots of fluorescence versus time. The slope of each plot was divided by the fluorescence corresponding to full hydrolysis, and multiplied by the substrate concentration to give velocity in micromoles per minute. Lineweaver–Burk plots (1/V versus 1/[S]) were linear for protease-degradable peptides, indicating Michaelis–Menten kinetic behaviour ( Supplementary Fig. 2 ). Kinetic parameters were determined by directly curve fitting plots of velocity versus substrate concentration to the Michaelis–Menten equation (to limit errors induced by Lineweaver–Burk double-reciprocal plots). Fluorescence did not increase over time for non-degradable peptides such that their kinetic parameters could not be determined. MePHA synthesis MePHA polymers were synthesized in a modular three-step process. First, MaHA was synthesized as previously described [41] . Briefly, Na-HA (90 kDa, Lifecore) was dissolved in DI H 2 O and a Dowex 50Wx8 ion-exchange resin was added and mixed at 600 r.p.m. for 5 h. The resin was filtered from the reaction vessel and the solution was titrated to pH 7.02–7.05 with tetrabutylammonium hydroxide (TBA-OH), frozen and lyophilized to yield HATBA. Next, HATBA was dissolved as a 2 wt% solution in anhydrous dimethyl sulfoxide (Fisher) and reacted with equivalent molar amounts of N-(2-aminoethyl)maleimide trifluoroacetate salt and BOP under N 2 for 4 h before dialyzing (8,000 MWCO, Spectra/Por) against cold DI H 2 O for 2 weeks. MaHA solutions were frozen, lyophilized and analysed via 1 H NMR to determine the degree of HA repeat functionalization with maleimide groups ( Supplementary Fig. 13 ). Although different degrees of maleimide functionalization were achieved (5–35%) all studies reported here were conducted with 10–15% functionalized MaHA (that is, 10–15% of HA repeats contain a maleimide linkage) for consistency between all materials. Second, thiolated peptides were synthesized as described above. Third, MaHA was dissolved as a 1 wt% solution in DI H 2 O and thiolated peptide fluorophore was stoichiometrically added such that thioether bonds would form in <6 maleimide repeats per HA polymer chain. About 90 kDa HA contains >230 repeat units on average such that 15% modified MaHA contains 35 maleimide repeats, of which <6 are consumed by thiolated fluorophore. After 30 min of mixing, MeP (protease degradable or non-degradable) was added in 1.4 times excess to maleimide groups and allowed to react for 4 h at room temperature to consume all remaining maleimide groups. The solution was titrated to neutral pH using 5 N sodium hydroxide, dialyzed against cold DI H 2 O for 72 h, frozen, lyophilized and stored at −20 °C. Final product conjugation was confirmed via 1 H NMR by the loss of maleimide peak and introduction of methacrylate peaks from the conjugated peptide ( Supplementary Fig. 14 ). Scaffold fabrication All degradation studies ( in vitro and in vivo ) were replicated ( n =3 or 4 as stated throughout) to determine statistical significance. Prior to any hydration step, all formulations of MePHA were sterilized under germicidal ultraviolet exposure for 45 min and maintained under sterile conditions thereafter. For rheological studies, solutions of 2 and 4 wt% MePHA with 0.05% Irgacure 2959 (I2959) in TTC buffer were exposed to 10 mW cm −2 of ultraviolet light (Omnicure S1000, 365 nm filter) for 15 min on an AR2000 stress-controlled rheometer (TA instruments; −20 mm diameter cone and plate geometry, 59 min 42 s cone angle and a 27 μm gap distance) under 0.1% oscillatory strain. To synthesize isotropic MePHA hydrogels for degradation studies, 50 μl solutions of 4 or 2 wt% MePHA with 0.05% I2959 in TTC buffer were added to a cylindrical mold (tip of a cut 1 ml syringe) and exposed to 10 mW cm −2 ultraviolet light for 15 min to induce gelation. To synthesize electrospun fibrous MePHA hydrogels, solutions of 1 wt% MePHA, 4.5 wt% PEO (900 kDa) and 0.05 wt% I2959 in TTC buffer were mixed at 110 r.p.m. for 24–48 h and loaded into syringes. These solutions were then electrospun onto a rotating mandrel (350 r.p.m. to maintain random fibre orientation during collection) in a custom environmentally regulated chamber (humidity 20–35%) with the following collection parameters: applied voltage: 21–26 kV, deflector voltage: 10–12 kV, collector voltage: −3 kV, distance from needle to collector: 18 cm, needle gauge: 18, flow rate: 1.0 ml h −1 . Multi-fibre electrospun mats used two separate syringes facing the rotating collection mandrel from opposite sides ( Fig. 5a ). To image electrospun fibrous MePHA hydrogels, fibres were collected onto aluminium foil and imaged with a FEI Quanta 600 environmental scanning electron microscope, or collected onto methacrylated coverslips [53] and imaged using confocal fluorescent microscopy (Zeiss Axio Observer Inverted microscope) or wide-field fluorescent microscopy (Olympus BX51). To crosslink electrospun MePHA hydrogels, dry scaffolds were exposed to 30 min of 10 mW cm −2 ultraviolet light under N 2 , swollen with 0.05% I2959 in TTC buffer and re-exposed to 10 mW cm −2 ultraviolet light for 1 min (thin films (10–30 μm) for confocal imaging—to limit photobleaching) or 20 mW cm −2 ultraviolet light for 30 min (for degradation studies). To determine fibre diameters, scaffolds were imaged in eight distinct scaffold areas and fibre diameters were quantified using ImageJ (>25 fibres per image, × 63 magnification—confocal, × 9500 magnification—SEM). Similar to the method previously described [54] , scaffold porosity was determined by converting confocal images ( × 63 magnification) of thin electrospun films to binary, thresholding the images and quantifying the void area of the image as a percentage of the total area (ImageJ, >6 images per condition). Unconfined compression testing was performed on swollen electrospun hydrogels using a TA Instruments DMA Q800 at constant strain rate of 10% per min. Compressive modulus was calculated from the slope of the stress–strain curve between 5 and 15% strain ( n =3). Degradation studies Isotropic hydrogels (50 μl) were equilibrated at 37 °C in 1 ml of TTC for 48 h in LoBind tubes and then placed into fresh sterile TTC buffer, 5 nM rhMMP-2 or sterile 1–500 U ml −1 Type II Collagenase (stock activity—335 U mg −1 ) in TTC buffer ( n =3 per condition). Units of activity are given by Worthington Biochemical COA and defined as ‘1 U liberates 1 μmol of L-leucine equivalents from collagen in 5 h at 37 °C, pH 7.5’. Fibrous hydrogels electrospun as thin films and thick mats (1 cm 2 area~1 mm thick dry) were equilibrated at 37 °C in TTC buffer for 48 h in a non-tissue culture-treated plate and then refreshed with TTC buffer, 10 nM rhMMP-2 (with 0.1 wt% reagent diluent to limit rhMMP-2 adsorption to well surfaces) or 5–500 U ml −1 Type II Collagenase in TTC buffer ( n =3, 4 per condition). Supernatant was collected and samples were refreshed with the corresponding media every 2 days to maintain enzymatic activity. Scaffolds not fully degraded at the end of studies were degraded in 1 mg ml −1 hyaluronidase to determine total HA content. The collected supernatant was analysed via fluorometric spectroscopy (FITC—excitation: 480 nm emission: 517 nm; RHO—excitation: 550 nm emission: 580 nm; Cyanine7.5—excitation: 788 nm emission: 818 nm) and compared with a standard curve of equivalent fluorescent MePHA. Individual scaffold degradation was formulated into a percentage and then averaged between groups to generate degradation profiles. Uronic acid (HA repeat units) release was quantified by colorimetric absorbance as previously described [55] to confirm degradation profiles observed by fluorescent MePHA release. To visualize degradation, thin film scaffolds were imaged with an Olympus BX51 microscope at different stages of degradation. Acquisition parameters (light intensity, camera exposure and resolution) were kept the same for all images to enable comparison between groups. Co-electrospun images were overlaid using ImageJ, again maintaining equivalent acquisition and processing parameters between compared images. Subcutaneous mouse model To evaluate in vivo degradation of electrospun fibrous hydrogels, 25 mm 2 scaffolds (MMP degradable or non-degradable, ~1-mm thick dry) conjugated with the GCKKG-Cyanine7.5 fluorophore (NIR) were equilibrated in sterile PBS for 48 h (37 °C) and then subcutaneously implanted into the dorsal region of adolescent BALB/C mice (male). Serial images were taken during a 6-week period using a LiCore live imaging system (800 nm), and signal intensity (photons per pixel per second) was measured by integrating equivalent areas over the region-of-interest. Quantified signal was normalized to peak intensity for individual scaffolds and then averaged to obtain degradation profiles for each scaffold ( n =4, 3 per condition). At the conclusion of the study, the tissue containing fibrous hydrogels was excised, fixed in formalin, embedded in paraffin, sectioned (5-μm slices) through the height of the scaffold region and stained with haematoxylin and eosin. The study adhered to the NIH Guide for the Care and Use of Laboratory Animals and was approved by the University of Pennsylvania's Institutional Animal Care and Use Committee. Statistical analysis All experimental data are reported as the mean of three or four individual samples. Single factor analysis of variances were performed for data sets with Tukey’s honest significant difference post-hoc testing and statistical significance was considered at P <0.05. How to cite this article: Wade, R. J. et al . Protease-degradable electrospun fibrous hydrogels. Nat. Commun. 6:6639 doi: 10.1038/ncomms7639 (2015).